Giant infrared absorption bands of electrons and holes in conjugated molecules Infrared (IR) absorption bands often convey identifying information about molecules, but are usually weak, having molar absorption coefficients <200 M −1 cm −1 . Here we report observation of radical anions and cations of conjugated oligomers and polymers of fluorene and thiophene that possess intense mid-infrared absorption coefficients as large as 50,000 M −1 cm −1 , perhaps the largest known for molecular species. For anions of fluorene oligomers, F n , n =2–4, IR intensities increase almost linearly with n , but with a slope much larger than one, indicating that the absorptions are not extensive properties. Large intensities seem to arise from a mechanism known for charged solitons and polarons in conjugated polymers. In this mechanism, vibrations of ungerade symmetry drive substantial displacements of charge, creating the large dipole derivatives responsible for intense IR absorption. Both experiments and calculations find that pairing with counter-ions attenuates IR band intensities. The IR bands may be diagnostic for bound ion pairs and their escape to form free ions. Infrared (IR) absorption by molecular vibrations can provide diagnostic structural and electronic information about molecules, but it is often weak; absorption coefficients, ε , in the mid-IR of >200 M −1 cm −1 are considered very strong. Stronger absorptions to ε =35,000 M −1 cm −1 are found for the C≡O stretching bands of metal hexacarbonyls [1] , [2] , [3] . These concur with the adage that bonds with substantial dipole moments tend to give strong IR absorption. Although such strong absorptions are rare in less polar bonds, Sakamoto et al. [4] reported IR absorption coefficients of 3,450 M −1 cm −1 for the radical anion of p -terphenyl and 7,820 M −1 cm −1 for the dianion. These do not come from vibrations of highly polar bonds. Similarly, early research on holes and electrons in conjugated polymers discovered vibrational absorption by ‘IR active’ molecular vibrations [5] , [6] , [7] , [8] , [9] . Extensive research on these ‘IRAV’ bands and Raman scattering in solid films of polymers and their ions [10] , [11] , [12] , [13] , [14] , [15] , [16] , [17] produced insight on the natures of the species and fascinating behaviour including possibly large intensities and Fano-like interferences. These are plausibly strong, but absolute intensities were not determined. The IRAV bands were interpreted with an amplitude theory [18] , [19] that has been further developed [20] along with related theories [21] , [22] , [23] including descriptions with a molecular viewpoint [24] , [25] . The present work takes advantage of ready determination of absolute IR absorption (extinction) coefficients in solution to find coefficients 10 times larger than that of Sakamoto et al. [4] 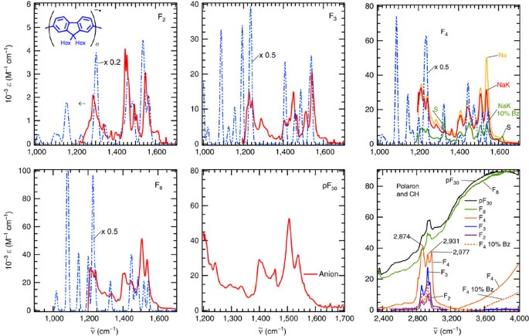Figure 1: IR absorption spectra of radical anions. IR spectra of oligofluorenes and a polyfluorene (Hex=n-hexyl) with an average length of 30 repeat units in THF-d8; the panels are labelled by the molecules from which the anions are formed. F4anions were produced under three conditions (see text). The experimental spectra are compared with computed spectra for ion pairs at 5 Å from the centre of the oligomer (blue dash-dot lines). The calculations give integrated intensities,A, (km mol−1). Each computed intensity has been replaced by a Gaussian of 20 cm−1full width at half maximum to estimate computed absorption coefficients, using the relationε=4.72A(see text). The computed intensities are scaled by factors indicated on the graphs. Bands labelled as S in the F4panel are imperfectly subtracted solvent absorptions. Incompletely subtracted solvent absorptions in the spectrum of F8−·in the last panel were corrected (seeSupplementary Fig. S5). IR spectra of anions Figure 1 displays IR spectra of radical anions of four fluorene oligomers and a polymer. In each case, the spectrum of the pure solvent (see Supplementary Figs S1 and S2 for solvent spectra) was subtracted from those of the samples containing the anions. Each of these molecules was reduced to make anions using NaK in deutereo tetrahydrofuran (THF- d 8 ). F 4 was also reduced in two other conditions. One was reduction by Na metal and the other was reduction by NaK in 90% THF- d 8 /10% benzene- d 6 . The spectrum with 10% benzene showed similar frequencies but substantially smaller absorption coefficients. In a similar solution with 20% benzene- d 6 (not shown), both frequencies and absorption coefficients were similar to those in 10% benzene. An expanded version of the F 4 anion graph is given in Supplementary Fig. S3 . The first five panels of Fig. 1 show mid-IR spectra from 1,200 to 1,700 cm −1 ; the sixth shows spectra of all the anions from 2,350 to 4,000 cm −1 . Strong solvent absorption precluded determination of spectra of the anions for frequencies <1,200 cm −1 and from 2,000 to 2,200 cm −1 . The region from 1,700 to 2,000 cm −1 is not shown because there was negligible absorption from the anions in the region. Concentrations of the anions were determined to be 0.27, 0.11, 0.4, 0.14 and 0.18 mM for F 2 , F 3 , F 4 , F 8 and pF 30 , respectively, based on measurements of visible bands ( Supplementary Fig. S4 ) in the solutions of anions and the known absorption coefficients of the anions [26] , [27] where determinations of absolute absorption coefficients were aided by the use of pulse radiolysis [26] . Figure 1: IR absorption spectra of radical anions. IR spectra of oligofluorenes and a polyfluorene (Hex= n -hexyl) with an average length of 30 repeat units in THF- d 8 ; the panels are labelled by the molecules from which the anions are formed. F 4 anions were produced under three conditions (see text). The experimental spectra are compared with computed spectra for ion pairs at 5 Å from the centre of the oligomer (blue dash-dot lines). The calculations give integrated intensities, A , (km mol −1 ). Each computed intensity has been replaced by a Gaussian of 20 cm −1 full width at half maximum to estimate computed absorption coefficients, using the relation ε =4.72 A (see text). The computed intensities are scaled by factors indicated on the graphs. Bands labelled as S in the F 4 panel are imperfectly subtracted solvent absorptions. Incompletely subtracted solvent absorptions in the spectrum of F 8 −· in the last panel were corrected (see Supplementary Fig. S5 ). Full size image The experimental spectra are compared with spectra computed by frequency calculations on the geometry-optimized anions in a polarized continuum model (PCM) reaction field simulating THF. The calculations used the ω PBE ( ω =0.1) functional that was found to give a good description of the optical transitions of anions of fluorene oligomers and the spatial extent of their polarons, which typically spread over four fluorene repeat units [26] . Computed IR bands in the CH stretch region (not shown) are small, and will be discussed below. Many or most of the anions are probably ion paired with K + , or possibly Na + counter-ions. Therefore, spectra were computed for ion pairs with Na + . Optimization of the positions of the Na + placed the Na + unreasonably close to the anions based on the computed optical spectra and energies. It is known that coordination of Na + or K + by THF causes these ions to pair more weakly with anions probably because the alkali ions surrounded by THF molecules act like much larger ions. The ion-pair calculations therefore optimized and computed IR spectra for anions with Na + counter-ions held at fixed, 5 Å, distances. This distance is between the ~2.5-Å distance of closest approach from optimizations and the 7–8-Å distance estimated for solvent-separated ions pairs [28] . As the actual distance is not known, these ion-pair calculations are provisional and are meant to illustrate trends. An example structure is shown in Supplementary Fig. S6 . The relation A (km mol −1 )=0.0106 ε w , where w is the full width at half maximum (FWHM) of the band in cm −1 is used in Fig. 1 to compare the computed integrated intensities A to observed spectra. This relation assumes that the bands are approximately Gaussian in shape. As bands often overlap, their widths are not precisely determined, but many of the widths appear to be ~20 cm −1 , giving ε =4.72 A. With this relation, the computed intensities were larger than experimental intensities. IR spectra of cations IR spectra of F 4 , F 8 and pF 30 produced by oxidation by nitrosonium hexafluorophosphate (NOPF 6 ) are shown in Fig. 2 . The CDCl 3 solvent permitted acquisition of spectra of the cations over a slightly larger frequency range. Absorption coefficients for the pF 30 cation were calibrated using ε (pF +· ) reported by Takeda et al. [27] For F 4 and F 8 cations, absorption coefficients of the visible bands were assumed to be similar to those of the corresponding anions [26] . We estimate that this approximation raises the uncertainty of the IR absorption coefficients of the cations to ±30%. The IR spectra of ion-paired cations used PF 6 − counter-ions. 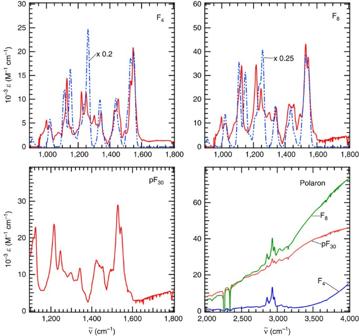Figure 2: IR spectra of positive ions. IR absorption spectra of radical cations created by NOPF6oxidation of F4, F8and pF30in CDCl3. Other experimental conditions are similar to those inFig. 1as are the calculations and their presentation (blue dash-dot lines). The calculations use PCM(CHCl3) with PF6−counter-ions at 5 Å. Figure 2: IR spectra of positive ions. IR absorption spectra of radical cations created by NOPF 6 oxidation of F 4 , F 8 and pF 30 in CDCl 3 . Other experimental conditions are similar to those in Fig. 1 as are the calculations and their presentation (blue dash-dot lines). The calculations use PCM(CHCl 3 ) with PF 6 − counter-ions at 5 Å. 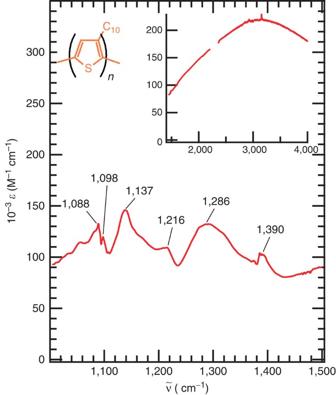Figure 3: IR spectra of a polythiophene cation. The IR absorption spectrum of P3DT+·in CDCl3under conditions as in those ofFig. 2. Full size image Figure 3 shows IR spectra of the cation of the polythiophene, poly(3-decylthiophene-2,5-diyl) (P3DT). P3DT +· was created by similar methods in CDCl 3 . Calibration of absorption coefficients used the result of Takeda and Miller [29] . In Fig. 3 , we see that the maximum of the polaron band is at ~3,000 cm −1 and that the band overlaps even the mid-IR vibrations from 1,000 to 1,400 cm −1 , which are broader than those of the fluorenes. Figure 3: IR spectra of a polythiophene cation. The IR absorption spectrum of P3DT +· in CDCl 3 under conditions as in those of Fig. 2 . Full size image The main features of the spectra of the ions are described here and discussed below after noting relations to known information: intensities of the main IR bands, expressed as molar absorption coefficients, are large, perhaps the largest we know of for any molecular species. The intensities for oligofluorene ions in Figs 1 and 2 depend strongly on length as seen in the plot of peak intensity in Fig. 4 and in Supplementary Fig. S7 , which plots intensities (extinction coefficients) integrated over four regions to sense averages over congested regions. Although this increase looks approximately linear from F 2 to F 4 , the slope is not unity: as the length doubles, the intensities of the bands shown increase by an average of a factor >7. The intensities level off for oligomers longer than F 4 , except for the CH stretch region, where intensities decrease. At high frequencies, usually ~2,000 cm −1 , broad continuous absorptions appear because of polaron bands that are well known for holes and electrons in conjugated polymers and oligomers. For the molecules studied here, the polaron bands were reported earlier in the near IR [26] , [27] , [29] . To estimate the IR intensities of CH stretches in Fig. 4 and Supplementary Fig. S7 , the absorption due to the polaron bands was subtracted using linear interpolation. Intensities of F 4 −· decreased by more than a factor of two on addition of a non-polar solvent, 10% benzene- d 6 . 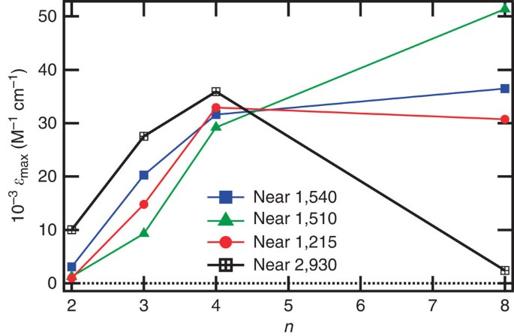Figure 4: Effect of length. Intensities at the peaks of four principal IR transitions in radical anions of fluorene oligomers, Fn, as a function of their lengths,n, in repeat units from experimental data inFig. 1. The actual peak positions vary slightly with the length of the oligomer. For example, the positions of the peak labelled as near 1,540 are at 1,549; 1,543; 1,540 and 1,538 cm−1forn=2,3,4 and 8. Computed spectra were in rough agreement with observed spectra, but for the most intense bands the computed frequencies often vary by up to 20% from the most intense observed frequencies. Agreement of computed frequencies with observed frequencies is best for F2−·and becomes poorer for longer oligomers. Figure 4: Effect of length. Intensities at the peaks of four principal IR transitions in radical anions of fluorene oligomers, F n , as a function of their lengths, n , in repeat units from experimental data in Fig. 1 . The actual peak positions vary slightly with the length of the oligomer. For example, the positions of the peak labelled as near 1,540 are at 1,549; 1,543; 1,540 and 1,538 cm −1 for n =2,3,4 and 8. Computed spectra were in rough agreement with observed spectra, but for the most intense bands the computed frequencies often vary by up to 20% from the most intense observed frequencies. Agreement of computed frequencies with observed frequencies is best for F 2 −· and becomes poorer for longer oligomers. Full size image IR spectroscopy has been shown to provide information about the nature of charge carriers in conjugated polymers [30] , and as discussed above, early research on holes and electrons in conjugated polymers discovered absorption by ‘IR active, IRAV’ molecular vibrations [5] , [6] , [7] , [8] , [9] . Although the absolute intensities of these IRAV bands were not determined, it is plausible that the IRAV bands have absolute intensities similar to those described here. The intensities found here are astonishing, raising the question why are they so strong? Theories of IR intensities [31] , [32] , [33] , [34] have evolved [23] , [24] , [25] to include contributions from two principal factors: dipole derivatives and proximity to electronic transitions. Substantial dipole derivatives arise when charge distributions evolve in response to vibrations [35] , [36] and these can become ‘massive’, for example, for charged solitons in polyacetylene [37] , [38] . The second contribution, to be discussed in connection with CH-stretching vibrations, arises from vibronic interactions with low-lying electronic transitions that enhance the dipole derivatives. Both factors are unusually effective in the conjugated ions studied here. We describe below how large dipole derivatives are enhanced for the C=C stretches and CH bends seen from 1,000 to 1,700 cm −1 , while interactions with electronic excitations seem to enhance CH-stretching intensities. For several of the vibrational modes in the 1,000–1,700 cm −1 region, vibrational displacement of the nuclei provokes a larger displacement of the polaron. This is seen in Fig. 5 , which displays the Kohn–Sham singly occupied molecular orbital (SOMO) computed for F 5 −· . The top panel shows the SOMO of the optimized (undisplaced) structure. The next panel shows the SOMO for structures stretched or compressed to the classical turning points of the 945 cm −1 vibration, where we observe a notable displacement of the SOMO bearing the charge. The stretch or compression of these structures produces dipole moments of 9.9 Debye in opposite directions: the charged polaron vibrates along with the molecular vibration producing big changes in dipole moment. This motion is more obvious in the large displacements of the SOMO with stretching or compression to five times the classical turning point, displayed in the lower panel of Fig. 5 . The mechanism giving ‘massive’ charge displacements for solitons [37] , [38] and for polarons [20] , [21] , [22] , [39] is pictorially described in Fig. 5 , and may resemble ‘the changes in electronic structures induced by specific vibrations’ mentioned by Sakamoto et al. 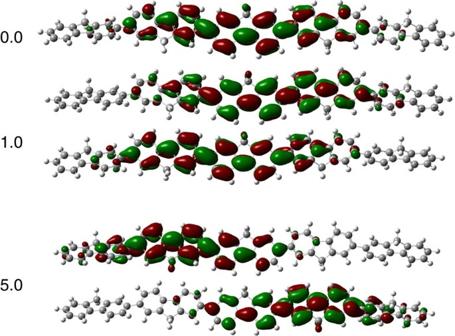Figure 5: Shift of charge on vibrational displacement. Kohn–Sham SOMO orbitals (3–21G,ωPBEω=0.1 in PCM for THF) in F5−·. At the top, labelled 0, is the SOMO of optimized F5−·. Next, labelled 1, are SOMOs from single-point calculations on structures stretched and compressed to the classical turning points of the 945 cm−1vibration. At the bottom, labelled 5, are SOMOs in similar structures displaced to five times the classical turning points. [4] Figure 5: Shift of charge on vibrational displacement. Kohn–Sham SOMO orbitals (3–21G, ω PBE ω =0.1 in PCM for THF) in F 5 −· . At the top, labelled 0, is the SOMO of optimized F 5 −· . Next, labelled 1, are SOMOs from single-point calculations on structures stretched and compressed to the classical turning points of the 945 cm −1 vibration. At the bottom, labelled 5, are SOMOs in similar structures displaced to five times the classical turning points. Full size image Figure 5 gives us a picture of polarons as objects that are not static. Instead, the polaron vibrates synchronously with several molecular vibrations. As for charged solitons [37] , [38] , an important feature to produce large IR intensities for the 945 cm −1 mode, discussed in Fig. 5 , and other bands giving large IR intensities, (for example, 1,038; 1,048; 1,142; 1,171; 1,217; 1,403; 1,487; and 1,517 cm −1 ) is that these vibrations are antisymmetric, transforming with the B representation in the C2 structure of F 5 −· . Supplementary Fig. S8 shows vector diagrams for displacements in these modes. Each of these modes that give high IR intensity contains displacements distributed along the length of the polaron. These modes comprise CH rocks and CC stretches along the axis of the molecule, so their displacements produce net displacement of the charge of the polaron. As for charged solitons [37] , [38] , they are ungerade: stretching of a bond on one side of the molecule is synchronous with compression of the symmetrically related bond on the opposite side of the molecule. The computed integrated intensity of the 945-cm −1 mode is A =131,877 km mol −1 . A somewhat similar, but symmetric (A) vibration at 995 cm −1 has an integrated intensity of only 1.3 km mol −1 . For such symmetric vibrations, charge on the left and right sides of the molecule both move towards the centre at the same time, so the polaron vibrates, but with no net change of dipole moment, and hence negligible IR intensity. For vibrations of appropriate symmetry, the frequency calculation in Gaussian 09, or other computational programs, captures the large dipole derivatives generated by this mechanism, yielding the large computed intensities. Exceptional dipole derivatives thus arise because the charge, self-localized in a polaron as illustrated in Fig. 5 , moves in response to a vibration with appropriate symmetry, generating a strong dependence of dipole moment on vibrational displacement. This effect is large when uncharged regions are present to the left and right of the polaron. Uncharged regions are seen at both ends in Fig. 5 , top panel. For ions of F 2 and F 3 , the polarons are confined by the short length of the oligomers, so less displacement of the polaronic charge occurs on vibration. As polarons in F n oligomers have a length of ~4.3 repeat units [26] , [27] , the IR enhancements are optimal at lengths slightly longer than four repeat units. For this reason, F 5 was chosen for the illustration in Fig. 5 . The mid-IR intensities in Fig. 4 increase approximately linearly with length for F n −· ( n =2–4). This increase begins at an intercept of zero intensity at n =1.9±0.1 repeat units (3.8 benzene rings). Thus, for molecules with lengths of <3.8 benzene rings, the intensities are small, but they increase rapidly above this length. The observed IR spectra of F 4 −· in Fig. 1 were strongest when F 4 was reduced by Na, weaker when reduction was by NaK and still weaker when 10% benzene- d 6 was added. As Na + is more strongly solvated [40] by THF than is K + , this order is consistent with weaker IR bands in (M + ,F 4 −· ) when the ion pairing is stronger. Computed IR spectra in Supplementary Fig. S9 predict that most IR bands are strongest in the free ion, and become weaker as the counter-ion is closer. Together, the experiments and calculations support the idea that ion pairing tends to decrease IR intensities. The calculations also predict that the positions of some IR bands shift with ion pairing and that some exceptionally large intensities will occur at frequencies below 1,100 cm −1 , especially in free ions (see also Supplementary Fig. S9 ). These calculated results are not tested for the anions in the present experiments because of solvent absorption. However, the region was observable for cations in CDCl 3 because of the good transparency of this solvent, and the observed absorption coefficients were not larger than those in other regions. The intensities were consistent with those computed for ion pairs (see Fig. 2 ). With the low dielectric constant ( ε =4.89) of chloroform, it is plausible that there are few free ions, and that the ion pairs are tightly bound. Quantum-chemical calculations often give good predictions of IR spectra for small molecules, including ions of terphenyl [4] , and even for charge-transfer salts [41] . The calculations reproduce some features of the observed spectra fairly well. However, they fail to predict bands observed near 1,300 cm −1 for F 3 −· and some predicted bands are too large, whereas others are too small. The calculations are somewhat better for fluorene cations in Fig. 2 . The failure of the calculations to give excellent descriptions of the observed spectra may arise because they are on optimized structures, each with a single conformation. The actual molecules almost certainly undergo conformational fluctuations, especially of dihedral angles between adjacent repeat units. The calculations do predict intensities to increase by factors of ~2 from F 2 −· to F 3 −· , but actual increases are much larger (see Fig. 4 ). This may signal that the range correction of the ω PBE functional does not fully predict the confinement of the charge in short oligomers. However, it may mean that ion pairing is tighter to the shorter F 2 −· , producing lower intensities; the calculations used a constant ion-pairing distance. The calculations also locate counter-ions 5 Å from the centre of the molecules, whereas the actual positions certainly fluctuate, possibly altering vibrational intensities. Supplementary Fig. S11 shows very substantial changes of a computed IR spectrum by movement of the counter ion. An accurate computational rendering is therefore likely to be challenging. The largest contrast between observed and computed intensities occurs in the CH-stretching region, 2,850–3,200 cm −1 . Observed bands reach absorption coefficients of nearly 10,000 M −1 cm −1 for F 2 −· and rise to ~40,000 M −1 cm −1 for F 4 −· . However, in the CH region the largest computed absorption coefficient for F 4 −· for the free ion is smaller by a factor of eight. For 5 Å ion pairs, the largest computed band is smaller by another factor of two. Supplementary Figs S10 and S11 give examples of the near absence of CH-stretching vibrations in a computed spectrum. This pattern holds for other ions; computed intensities are much smaller than those observed. Supplementary Fig. S12 displays displacement vectors for two of the CH-stretching vibrations giving the largest computed IR intensities. All the CH-stretching vibrations are localized, as are the two in Supplementary Fig. S12 , and for most their displacements are in nodal planes of the π electrons. Such vibrations are expected to produce only small dipole derivatives, consistent with the computed results. The fact that large CH bands are observed despite weak expected and computed dipole derivatives might be understood on the basis of enhanced IR intensities due to vibronic coupling [4] , [17] , [20] , [24] , [25] , [39] to low-energy electronic excited states. Nafie’s [25] description for the transition dipole of an IR band at frequency ω a multiplies the contributions of dipole derivatives to transition moments by a term LL e describes contributions from each electronic transition at frequency ω eg 0 . When all electronic excitations lie much higher than the vibrational excitation ( ω eg 0 >>ω a ), dipole derivatives are amplified little by electronic excitations. It is apparent in Figs 1 , 2 , 3 that the P 1 transitions of polarons [24] , [25] provide low-lying electronic states at energies near to those of the CH vibrational transitions that could amplify their IR intensities. The intensities computed here ( Figs 1 and 2 , Supplementary Figs S9 and S11 ) for the CH vibrations are much weaker than the observed CH bands, possibly because vibronic coupling to excited states is not yet incorporated into Gaussian 09 for calculation of IR intensities. Equation (1) estimates enhancements of 1.7, 1.4 and 1.3 for 3,100 cm −1 bands in anions of F 4 , F 3 and F 2 . These small enhancements, based on maxima of the P 1 polaron bands, are well below what is needed to understand the large observed CH bands, but it is conceivable that the fluctuating polarons can give very small denominators in equation (1) and thus much larger enhancements. Although the polaron band enhances intensities of CH vibrations, there can be too much of a good thing. In the CH regions of F 8 −· and pF 30 −· ( Fig. 1 ) and F 8 +· and pF 30 +· ( Fig. 2 ) the broad, continuous polaron bands are not just near the CH vibrations but overlap them. Instead of producing still larger intensities from the CH vibrations, this overlap with the polaron bands seems to reduce their intensities relative to those in F 4 −· or F 4 +· . This interesting effect could provide clues as to the nature of the broad polaron absorption bands. For P3DT +· ( Fig. 3 ), the polaron absorption extends to such low energies that the overlap and loss of intensity occurs even for the mid-IR vibrations, which appear to be broadened and of lower intensity. This behaviour and related anti-resonances [20] can be understood in terms of amplitude theory [18] , [20] , [21] , [22] , [39] or the theory of Nafie [25] , which predicts intensity enhancement from a larger positive dipole matrix element when the low-lying electronic state is above the vibrational excited state ( ω eg 0 > ω a ) but a negative matrix element when ω eg 0 < ω a . If both occur simultaneously, interference (cancellation) can occur, but simultaneity is important because, as Nafie notes, the dipole strength is the ‘absolute square of the electric–dipole transition moment, always a positive quantity.’ Interference between contributions from polaron states above and below the vibrational quantum could explain the lower intensities when the polaron bands overlap the vibrations. This would require that the polaron bands are homogeneously broadened, at least on the timescale of vibration. In conclusion, extremely intense mid-IR bands were observed to arise from molecular vibrations in conjugated oligomers and polymers. These intense bands occur only in molecules containing electrons or holes (radical anions or cations), not in neutrals. Intensities of these IR bands are competitive with the largest IR absorption coefficients measured for molecular species. They are smaller in short oligomers and increase with length of the oligomer until the oligomer becomes longer than the length of the polaron. The IR absorption bands are similar or identical to ‘IR active, IRAV’ bands observed in polymer films. Intensities of the IRAV bands have not been reported, but it is likely that they are similar to those determined here. Explanations for the astonishing intensities seem to lie in the properties of polarons, which undergo motions in response to molecular vibrations having appropriate symmetry. For F 5 −· , these are vibrations transforming with B representations in C2 symmetry. These vibrational motions drive the polaron along the long axis of the conjugated molecule generating large dipole moments as discussed earlier for charged solitons and polarons [18] , [20] , [21] , [22] , [37] , [38] , [39] . The present findings indicate that polarons in conjugated chains are dynamic, undergoing changes of charge density driven by molecular vibrations. Density functional theory calculations gave a fair, although not excellent, description of the frequencies and intensities. Experiments and calculations together point to a substantial sensitivity of the IR bands to ion pairing: Measurement of IR bands during charge separation may have the potential to distinguish ion pairs from free ions, possibly even distinguishing intermediates in the charge escape process. The second mechanism producing large IR intensities involves vibronic interaction of vibrations with low-lying electronic states. Here the vibrational transitions borrow intensity from low-energy transitions of polarons. Chemicals Regioregular P3DT (Rieke Metals, Inc., >98.5% head-to-tail) was purchased from Aldrich and used without further purification. Gel permeation chromatography measurements revealed a number-averaged molecular weight M n ≈38,000 and a weight-averaged molecular weight M w ≈120,000 g per mole (polydispersity index M w / M n ≈3.2) [29] . From the measured M n , the average number of units is estimated to be n ~170. The syntheses and characterization of oligofluorenes (F) and polyfluorene (pF 30 ) were reported previously [42] . The obtained pF was fractionally separated with preparative scale gel permeation chromatography to provide samples with different average lengths. The polydispersity of the pF 30 used here was 1.82. Sodium potassium alloy from Aldrich and NOPF 6 from Alfa-Aesar were used as received. The molecules under study were reduced or oxidized in deuterated THF or chloroform. These liquids were able to dissolve the molecules and had reasonably good IR transmission. Their spectra and those of some other solvents are shown in Supplementary Figs S1 and S2 . THF- d 8 (Aldrich, anhydrous, inhibitor free) was stirred with sodium potassium alloy for several days, vacuum distilled from sodium potassium alloy and stored under argon. Deutereo chloroform (Aldrich, HPLC grade, stabilized with aluminium metal) was treated repeatedly with 5 Å molecular sieves and stored under argon. Chemical reduction and oxidations All reductions and oxidations have been conducted inside an inert atmosphere glovebox. Oligomers (F n ) and polymers (pF and P3DT) were reduced with sodium potassium alloy (NaK) in THF- d 8 . F 4 was also reduced by Na metal chunks, but the reaction with Na metal took a few days to obtain sufficient concentration of anion for IR studies. Oxidations were carried out heterogeneously with NOPF 6 in deutereo chloroform. Both reactions were monitored with ultraviolet–visible-near IR in a 1.0 or 0.5-mm path length dry quartz optical cell. Concentrations of anions were determined from the absorptions ( Supplementary Fig. S3 ) along with known absorption coefficients [26] , [27] , [29] . Care was taken to add one or less reducing or oxidizing equivalent to each oligomer, or for polymers, to produce polarons well spaced from each other in the polymer chains. Absorption coefficients of pF anions and cations are similar [27] . For cations of fluorene oligomers, the absorption coefficients are not known but were estimated to be similar to those of the corresponding anions. IR spectroscopy IR spectroscopy was carried out in a gastight Harrick Scientific demountable liquid transmission cell (DLC-S25) constructed from a chemically inert stainless steel body. Two ports with Swagelok fittings permit static and flow experiments. The two CaF 2 windows used are separated with PTFE spacers; a 0.95-mm spacer was used in the present experiments. For sample preparation, the cell was filled in the glovebox by injecting the reactive cation or anion solution through one port. The cell was rinsed twice with the reduced or oxidized solution; the spectrum was taken from the third filling. The two ports were closed tightly with Swagelok caps and the cell transported in ambient air to a Thermo Scientific Nexus 670 FTIR spectrometer where the IR spectrum was recorded within 10 min. Fourier transform infrared spectra were recorded at 2 cm −1 spectral resolution with the Happ–Genzel apodization function and two levels of zero filling. Spectra of the anions in the sealed cell were typically stable for an hour with the cell surrounded by air, but some possible loss contributed to the uncertainty of the reported absorption coefficients, which we estimate to be ±20%. Density functional theory computations Density functional theory computations were carried out with Gaussian 09, C.01 (ref. 43 ). Frequency calculations were performed after optimization of geometries, both using the ω PBE long range-corrected functional [44] , with ω =0.1, and the PCM reaction field to simulate solvation in either THF or chloroform. Vibrational frequencies were unscaled. The reported results used the 3–21 g basis set. Tests with 6–31 g* calculations produced only small differences as did tests with the SMD reaction field. Depictions used GaussView 5. How to cite this article: Zamadar, M. et al. Giant infrared absorption bands of electrons and holes in conjugated molecules. Nat. Commun. 4:2818 doi: 10.1038/ncomms3818 (2013).